Coherent dynamics of a telecom-wavelength entangled photon source Quantum networks can interconnect remote quantum information processors, allowing interaction between different architectures and increasing net computational power. Fibre-optic telecommunications technology offers a practical platform for routing weakly interacting photonic qubits, allowing quantum correlations and entanglement to be established between distant nodes. Although entangled photons have been produced at telecommunications wavelengths using spontaneous parametric downconversion in nonlinear media, as system complexity increases their inherent excess photon generation will become limiting. Here we demonstrate entangled photon pair generation from a semiconductor quantum dot at a telecommunications wavelength. Emitted photons are intrinsically anti-bunched and violate Bell’s inequality by 17 standard deviations High-visibility oscillations of the biphoton polarization reveal the time evolution of the emitted state with exceptional clarity, exposing long coherence times. Furthermore, we introduce a method to evaluate the fidelity to a time-evolving Bell state, revealing entanglement between photons emitted up to 5 ns apart, exceeding the exciton lifetime. An optical network of remote quantum computers offers the potential for distributed quantum computing [1] , with individual nodes based on a range of quantum computer architectures such as linear optics [2] , ions [3] , [4] or electron spins [5] . However, successful distribution of photonic qubits depends on availability of suitable high-fidelity sources for links. Most experiments involving the distribution of entanglement over fibre have used downconversion as the source of entangled photons [6] , [7] , [8] , [9] , [10] , [11] . The Poissonian emission statistics of such systems produces an increasing number of multiple pairs as the generation probability increases [12] , and the probability of generating multiple pairs simultaneously is proportional to the probability of generating two single pairs separated by a chosen time, irrespective of pump power. There is therefore motivation to develop quantum light sources at telecom wavelengths that emit no more than one entangled photon pair per cycle. Semiconductor quantum dots are a promising platform for single [13] , [14] , [15] , [16] , [17] , [18] and entangled photon emitters [19] , [20] , owing to fundamentally sub-Poissonian emission statistics and common features with standard optoelectronics such as electrical control and pumping. So far, most progress has been made at shorter wavelengths around 900 nm, unsuitable for transmission over long distances in fibre. Furthermore, for optical quantum circuits based on dielectric waveguides or photonic crystals, losses can be reduced by using longer wavelengths owing to a larger ratio between the microstructure’s dimensions and size of fabrication imperfections. Entangled photons are generated by the radiative cascade of the biexciton state via the exciton state to the ground state [19] , [20] . The fine-structure splitting of the orthogonally polarized exciton photons [21] is caused by asymmetries of the quantum-dot crystal structure, and must be small compared with the spectral bandwidth of the photons [22] , or frequency bandwidth of the detectors [23] , to allow entanglement to be discerned. Minimizing the splitting is typically achieved by growing quantum dots at a particular wavelength, ~885 nm, due to a relationship between splitting and emission energy [24] . Thus realization of a telecommunication wavelength quantum-dot-entangled light source is especially challenging, as increasing the wavelength also increases the splitting, allowing only classical correlations to be observed [25] . In our approach (detailed in the Methods), telecommunication-wavelength emission is achieved by combining InAs quantum dots with an additional InGaAs strain relaxation layer to increase the emission wavelength. Despite the relatively weak confinement in the growth direction afforded by the 2D InGaAs layer, we show this arrangement embedded within a p-i-n diode supports sufficiently high electric fields to drastically reduce the fine-structure splitting, allowing emission of entangled photon pairs to be detected. Control and evolution of exciton states Photoluminescence of a device is shown in Fig. 1a as a function of internal electric field. The biexciton (XX) and exciton (X) transitions tune smoothly with electric field owing to the quantum-confined Stark effect, and remain within the telecommunications wavelength O band for fields>180 kV cm −1 . 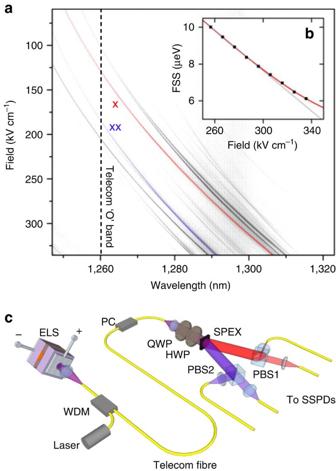Figure 1: Device characteristics and system setup. (a) Stark shifts of the various excitonic emission lines are shown. The exciton emission (X) has been artificially coloured red and the biexciton line blue (XX). The shorter wavelength lines visible at the higher internal fields are likely to be excited states of the quantum dot. (b) Variation of the fine-structure splittingδ(FSS) with internal electric field. Points are experimental measurements, red line is a hyperbolic fit and grey line is the linear component of the fit. (c) Schematic diagram of the experimental arrangement including an entangled light source (ELS), wavelength division multiplexer (WDM), polarization controller (PC), rotatable quarter-wave plate (QWP) and half-wave plate (HWP), spectrograph (SPEX), polarizing beam splitters (PBS1 and 2) and superconducting single-photon detectors (SSPDs). Figure 1b shows the variation of the fine-structure splitting with electric field. The splitting reduces hyperbolically with increasing electric field, becoming significantly nonlinear close to the minimum splitting of ~6 μeV, as shown by the fitted red line [26] . In all other quantum dots with neutral exciton and biexciton transitions, splitting reduced with increasing electric field. Figure 1: Device characteristics and system setup. ( a ) Stark shifts of the various excitonic emission lines are shown. The exciton emission (X) has been artificially coloured red and the biexciton line blue (XX). The shorter wavelength lines visible at the higher internal fields are likely to be excited states of the quantum dot. ( b ) Variation of the fine-structure splitting δ (FSS) with internal electric field. Points are experimental measurements, red line is a hyperbolic fit and grey line is the linear component of the fit. ( c ) Schematic diagram of the experimental arrangement including an entangled light source (ELS), wavelength division multiplexer (WDM), polarization controller (PC), rotatable quarter-wave plate (QWP) and half-wave plate (HWP), spectrograph (SPEX), polarizing beam splitters (PBS1 and 2) and superconducting single-photon detectors (SSPDs). Full size image Following emission of the biexciton photon, conservation of angular momentum dictates that the spin-state of the remaining single exciton will be entangled with the polarization of the biexciton photon. For finite fine-structure splitting, δ , the two eigenstate components of the single exciton state will then evolve, picking up a phase difference δt /ħ over time t until the exciton photon is emitted [23] . The corresponding two-photon evolving Bell state is as follows. Here subscripts identify the biexciton and exciton photons, and H and V are the horizontal and vertical linear polarizations aligned with the eigenstates of the quantum dot. Measurement of a biexciton photon in a H or V eigenstate projects the exciton into a static polarization correlated state. In contrast, measurement of a biexciton photon superposition state with polarization collapses the exciton photon into a state with evolving polarization , which rotates around the equator of the Poincaré sphere as shown in Fig. 2a by the blue arrow. The fraction of the exciton photon state copolarized with the detected biexciton photon thus oscillates with time delay according to cos 2 ( δt /2ħ− φ ), that is, with constant frequency but phase dependent on the polarization basis. 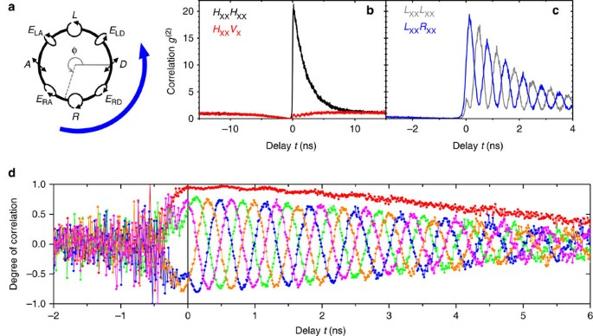Figure 2: Correlations between polarization states. (a) Expected evolution of the exciton polarization state represented on a Poincaré sphere. The exciton (X) state, initialized by measurement of the biexciton (XX) state, evolves with time around the equator as indicated by arrows. (b,c) The black (red) lines show correlation data for parallel (orthogonal) rectilinear polarizations and the grey (blue) lines show parallel (orthogonal) circular polarizations in the detection system basis. (d) The degree of correlation calculated for rectilinearH–V(red), diagonalD–A(green), circularL–R(blue), ellipticalELD–ERA(orange) and ellipticalELA–ERD(magenta) detection system bases. Figure 2: Correlations between polarization states. ( a ) Expected evolution of the exciton polarization state represented on a Poincaré sphere. The exciton (X) state, initialized by measurement of the biexciton (XX) state, evolves with time around the equator as indicated by arrows. ( b , c ) The black (red) lines show correlation data for parallel (orthogonal) rectilinear polarizations and the grey (blue) lines show parallel (orthogonal) circular polarizations in the detection system basis. ( d ) The degree of correlation calculated for rectilinear H – V (red), diagonal D – A (green), circular L – R (blue), elliptical E LD –E RA (orange) and elliptical E LA –E RD (magenta) detection system bases. Full size image Photon pair correlations and entanglement Polarization-dependent correlations are measured for emitted photon pairs under continuous-wave (cw) optical excitation, using telecommunications fibre and the system shown schematically in Fig. 1c (Methods). The polarization measurement basis is set jointly for both the XX and X photons with shared optics, and time-dependent correlations are recorded for co- and cross-polarized photon pairs. Such measurements of pairs of photons only in the same polarization bases can determine the majority of elements in a two-photon density matrix, including all those required to determine the fidelity with the Bell states, as we discuss below. Figure 2b shows correlations measured in the rectilinear { H , V } polarization basis. For coincident photon pair detection at t =0, copolarized detection is dominant, consistent with the expected Bell state. The intensity of the peak decays for small positive delays due to the finite X lifetime and, to a lesser extent, re-excitation. For small negative delays, the photon-pair intensity drops close to zero indicating exciton photons are emitted following biexciton photons and not before, as expected from the radiative decay process crucial to entanglement creation. Second-order correlation measurements of the individual X and XX photon streams reveal highly sub-Poissonian statistics, with measured g (2) (0) of 7.4 and 13.7% without compensation for detector jitter. Figure 2c shows correlations in the circular basis consisting of left (L, φ = π /2) and right (R, φ =3 π /2) hand polarizations. High-visibility multiple oscillations are observed with increasing time delay, as the exciton photon polarization evolves as described above. The degree of correlation, C , describes the contrast between co- and cross-polarized correlations in a given basis, and is plotted in Fig. 2d . For the rectilinear basis shown in red, C begins close to unity and decays smoothly and slowly predominantly due to re-excitation. For the circular basis, shown in blue, C oscillates with the predicted cosine form [23] , [27] . The degree of correlation is also shown measured in the diagonal (green) and two elliptical bases (magenta and orange) that complete an equally spaced set around the equator of the Poincaré sphere. All traces show remarkably similar oscillations, differing only by the initial evenly spaced phase φ as expected. In order to prove the emission from our device is entangled, we determine the entanglement fidelity. To begin, we introduce a method to extract the fidelity to the expected ideal evolving state directly from our measurements. In Supplementary Note 1 , we show that the fidelity F ( t )=‹ Ψ B ( t )| ρ | Ψ B ( t )›, where ρ is the emitted two-photon density matrix, is where the time-dependent polarization correlations coefficients C are measured in the rectilinear ( HV ), circular ( LR ), diagonal ( DA ) and elliptical ( E LD −E RA and E LD −E RA ) polarization bases as denoted by subscripts (see Supplementary Note 1 ). The fidelity to various static Bell states is determined by substituting δt /ħ for the static phase between | H XX H X › and | V XX V X ›, reducing it to the widely used expression [22] F + =[1+ C HV + C DA − C LR ]/4 in the case of the Bell state . The fidelity to four static Bell states is shown in Fig. 3a . In each case the fidelity peaks above 0.8, and oscillates sinusoidally, with initial phase determined by the reference state. We now evaluate the fidelity of the emission to | Ψ B ( t )› for any time delay as shown by the thick grey line in Fig. 3a and separately in Fig. 3b for the fitted fine-structure splitting of δ =6.14±0.02 μeV. The fidelity to the time-evolving Bell state decays smoothly towards 0.25, the value for uncorrelated states, once emission due to re-excitation of the dot dominates. The fidelity remains above 0.5, the maximum level expected for any classical photon-pair source, for ~5 ns corresponding to ~7 evolution periods of the single exciton state. 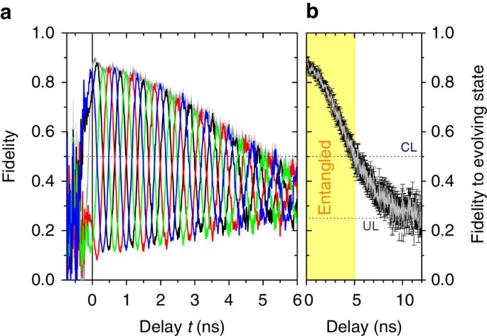Figure 3: Fidelity of entanglement. (a) Black, green, red and blue lines show measured fidelity to static entangled states (|HH›+exp(iπn/2)|VV›)/√2, wheren={0,1,2,3} ,respectively. The grey line indicates the fidelity to the time-evolving entangled state and is plotted by itself in (b) for clarity. The levels indicated are the classical limit (CL) and the uncorrelated level (UL). The yellow region indicates the times for which the fidelity exceeds the classical limit, and emission is entangled. Error bars are ±1 s.d. and are derived from counting statistics. Figure 3: Fidelity of entanglement. ( a ) Black, green, red and blue lines show measured fidelity to static entangled states (| HH ›+exp(i πn /2)| VV ›)/√2, where n ={0,1,2,3} ,respectively. The grey line indicates the fidelity to the time-evolving entangled state and is plotted by itself in ( b ) for clarity. The levels indicated are the classical limit (CL) and the uncorrelated level (UL). The yellow region indicates the times for which the fidelity exceeds the classical limit, and emission is entangled. Error bars are ±1 s.d. and are derived from counting statistics. Full size image Bell’s inequalities [28] are arguably the best-known entanglement tests and useful indicators of device suitability for applications that demand stronger entanglement, such as quantum key distribution [29] . Bell measurements are also sensitive to the measurement basis of the particular inequality formalism, usually selected to optimally exceed the classical limit of 2. For the evolving entangled state observed here, we therefore present a time-dependent formalism of Bell’s parameter S B derived from an evolving optimal CHSH [30] -type Bell inequality ( Supplementary Note 1 ). 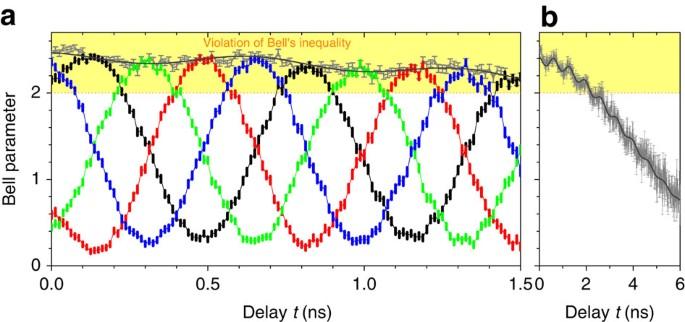Figure 4: Bell Parameter tests. (a) Coloured lines show Bell parameter tests optimized for the static entangled states inFig. 3a. Light grey line shows measured continuous violation of Bell’s inequality optimized for the evolving entangled state. Dark grey line is corresponding fitted behaviour. (b) Bell’s parameter for an evolving entangled state in (a) shown and fitted over a larger time range. Yellow regions represent regions where Bell’s inequality is violated. Symbol heights and error bars represent ±1 s.d. and are derived from counting statistics. Conveniently, this may be expressed in terms of the correlation coefficients C as follows; Figure 4a shows four static Bell parameters arising from combinations of the rectilinear degree of correlation with each of the other four basis sets, derived by substituting δt /ħ with a fixed phase into S B ( t ) ( Supplementary Note 1 ). As the Bell state evolves, the optimal Bell measurement rotates and each of the Bell parameters corresponds to an optimal measurement at different phases of the evolution. Throughout the evolution cycle, emission violates Bell’s inequality according to one of the Bell tests, although each individual Bell test is violated for just over 1/4 of a cycle each. In contrast, oscillations in Bell’s parameter are almost eliminated for an evolving Bell test, shown in grey, and continuous violation of Bell’s parameter for an evolving entangled state is reported. The observed maximum of 2.53±0.03, and the average over the first 100 ps of 2.49±0.03 both exceed the classical limit by 17 s.d. Figure 4: Bell Parameter tests. ( a ) Coloured lines show Bell parameter tests optimized for the static entangled states in Fig. 3a . Light grey line shows measured continuous violation of Bell’s inequality optimized for the evolving entangled state. Dark grey line is corresponding fitted behaviour. ( b ) Bell’s parameter for an evolving entangled state in ( a ) shown and fitted over a larger time range. Yellow regions represent regions where Bell’s inequality is violated. Symbol heights and error bars represent ±1 s.d. and are derived from counting statistics. Full size image We note that some weak residual oscillations may be discerned in the evolving Bell test results, more clearly shown over longer time periods as revealed in Fig. 4b . Their origin is deviation between the entangled state emerging from the fibre and the reference evolving Bell state probed using our measurement system, which can reduce Bell’s parameter with periodicity governed by the fine-structure splitting. We can analytically show that a small deviation of the eigenstates’ polarization basis from rectilinear reproduces observed behaviour very well, when combined with the Gaussian decay. Fits to the data shown in Fig. 4a and independently over a larger time range in Fig. 4b are shown as dark grey lines (see Methods), and agree with our data within the estimated error. The maximum of Bell’s parameter extracted from the fits is 2.47±0.01. Photon pair coherence To eliminate uncorrelated photon emission from re-excitation and reveal the coherence of the photon-pair state, correlation measurements were performed under pulsed laser excitation (Methods). The degree of correlation is plotted in Fig. 5a , which shows slowly decaying oscillations extending many times beyond the ~4 ns exciton radiative lifetime, extracted from the exponentially decaying biphoton intensity plotted in Fig. 5b . We fit the exponentially decaying amplitude of oscillations in the degree of correlation, as shown by the red lines, and determined the photon-pair coherence time to be 17.9 ns, over four times the exciton radiative lifetime, and significantly longer than that observed in cw experiments above owing to suppression of re-excitation. The long photon-pair coherence time is attributed to its inherent robustness against common sources of dephasing. For example, local charge fluctuations electrostatically perturb the H and V exciton eigenstates almost equally, leading to a negligible change in their phase difference. In contrast, first-order coherence times of the individual photons are sensitive to the overall phase changes caused by such fluctuations, causing dephasing within a few hundred picoseconds. 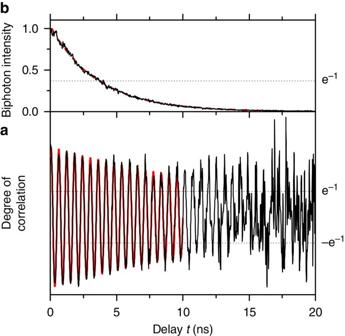Figure 5: Coherence of evolving entangled state. (a) Degree of correlation for the device under pulsed excitation shown as a black line (Methods). Red line is a numerical fit with coherence time 17.9 ns. (b) Normalized photon-pair intensity as a function of delayt, indicating far shorter radiative decay time of <4 ns. Figure 5: Coherence of evolving entangled state. ( a ) Degree of correlation for the device under pulsed excitation shown as a black line (Methods). Red line is a numerical fit with coherence time 17.9 ns. ( b ) Normalized photon-pair intensity as a function of delay t , indicating far shorter radiative decay time of <4 ns. Full size image The remaining observed weak decay of the photon-pair coherence may be attributed to incoherent refilling from nearby trapping centres or time-averaged coherent variation of the fine-structure splitting due to nuclear-spin fluctuations [31] . For the latter, we numerically estimate that the observed photon-pair coherence time can be reproduced by fluctuating nuclear hyperfine interactions with s.d. 1.0 μeV, similar in magnitude to reported values for other InGaAs quantum dots. The reported generation of entangled photon pairs at a telecommunications wavelength, and transmission over a standard single-mode optical fibre, represents an important step towards real-world applications in quantum networks. New analysis has introduced fidelity and Bell parameter measurements for an evolving entangled state with continuous high fidelity (up to 85%) and strong inequality violation (by ~17 s.d.) over multiple periods of evolution of the exciton state. Further exploration of quantum-dot growth conditions and techniques may further reduce the minimum fine-structure splitting and the field required to achieve it, and the potential to electrically excite our device [32] has strong practical appeal. Sample structure The sample was grown by molecular beam epitaxy on a GaAs substrate. The InAs quantum-dot layer was located in a quantum well within the intrinsic region of a p-i-n diode containing a weak planar cavity comprising AlGaAs/GaAs distributed Bragg reflectors to help couple photons out of the device. The InAs dot layer was deposited 5 nm above a short-period superlattice equivalent to Al 0.75 Ga 0.25 As and was capped with a 5 nm nominally In 0.23 Ga 0.77 As strain-relaxing layer and a further 10 nm of GaAs before a second similar superlattice barrier. Wafer material was annealed for ~6 min at ~650 °C to reduce the typical quantum-dot emission wavelength by ~40 nm before electrically contacted devices were fabricated. An array of apertures in an evaporated aluminium layer on the surface of the device provided the ability to optically address single quantum dots. The internal electric field was estimated as the built-in potential of the AlGaAs barrier (taken to be 2.2 V) minus the applied bias voltage divided by the width of the intrinsic region (203 nm). Quantum dots were studied with wavelength within the range 1,250–1,340 nm, which loosely corresponds to the bandwidth of the optical cavity. The dot selected for this study has attributes not uncommonly found within the population of 40 quantum dots with identifiable line structure characterized. Experimental arrangement The experimental arrangement is shown schematically in Fig. 1c . The sample was operated at ~17 K and emission was coupled at low temperature into standard SMF-28 optical fibre. The fine-structure splitting was used to set a polarization controller in order to map emission from the eigenstates of the dot close to (within around 9° on the Poincaré sphere) the basis states of the polarization selection system. We refer to these states as H and V , the horizontal and vertical states of the measurement system. Polarization state transformation by a quarter- and a half-wave plate in series followed by spectral separation of the exciton and biexciton emission using a diffraction grating and polarization selection by polarizing beam splitters was performed in free space. This ensured that the relationships between measurements in different polarization states were well known. One biexciton and two exciton optical signals were coupled back into optical fibre and delivered to commercial superconducting niobium nitride nanowire single-photon detectors with pairwise timing jitter of ~100 ps. Similar results were achieved by selecting either of the orthogonal biexciton states consistent with an unpolarized source. This measurement, and the pulsed results were measured independently from the other entanglement experiments presented here. Count rates were a few tens of kHz, strongly limited by the low excitation rates selected to reveal the time-dependent physics of our system. We estimated that emission was collected with an efficiency ~1%, based on the excitation rate, estimated losses after the collection lens, and detection rate of cw excited X photons. The statistics of the delays between detection events in pairs of detectors were recording using time-to-amplitude convertors. No attempt was made to map diagonal or circular emission from the dot to the corresponding states of the detection system so an arbitrary rotation about the H / V axis of the Poincaré sphere existed between polarization states of the dot and detection system. The measurement basis states of interest were cycled through repeatedly during an entanglement measurement to confirm that the polarization state evolution in the fibre was stable to within ~3° over the entanglement measurement. Errors on g (2) correlations were determined from Poissonian counting statistics, which were propagated to provide error estimates for degree of correlation, and various expressions for fidelity and Bell’s parameters. Time-evolving bell parameter analysis Fits to the time-evolving Bell parameter measurements shown in Fig. 4 were achieved using the product of a Gaussian and the function , which is the expected value when the polarization eigenbasis of an entangled evolving Bell state differs from the state probed by the measurement of a small latitudinal angle α and longitudinal angle β on the Poincaré sphere. The fine-structure splitting δ was not fitted, but fixed to the experimentally determined value. Photon-pair coherence analysis The photon-pair coherence measurements presented in Fig. 5 were performed at −4.2 V bias with a 1,064-nm ps-pulsed diode laser at a deliberately slow repetition rate of 20 MHz, selected in order to reveal time-dependent processes such as photon-pair decoherence, which occurs on a timescale of several 10 s of ns. Though weak emission intensity prevents precise fits for large times, good fits of exponentially decaying oscillations are achieved to the first 10 ns of data, allowing the coherence time to be estimated. For other quantum dots with significantly shorter radiative lifetimes, it will be possible to perform all correlation measurements in a pulsed mode using a higher repetition rate at the expense of obscuring the slow time-dependent effects. The magnitude of the nuclear-spin fluctuations required to reproduce the observed decoherence was determined following Stevenson et al . [31] and the procedure is summarized as follows. The nuclear-spin configuration within the quantum dot creates an effective magnetic field S c /μ B g , which interacts with the exciton to increase the fine-structure splitting to and introduce partial circular polarization to the eigenstates. The corresponding two-photon density matrix is weighted and integrated with respect to a normally distributed S c with mean 0 and s.d. σ . Using the measured value for δ , σ was fitted numerically to reproduce the experimentally measured decay in amplitude of second-order correlations. Supplementary information accompanies this paper at http://www.nature.com/nature communications How to cite this article: Ward, M. B. et al. Coherent dynamics of a telecom wavelength-entangled photon source. Nat. Commun. 5:3316 doi: 10.1038/ncomms4316 (2014).